In-situ formation of one-dimensional coordination polymers
              in molecular junctions We demonstrate the bottom-up in-situ formation of organometallic
                oligomer chains at the single-molecule level. The chains are formed using the
                mechanically controllable break junction technique operated in a liquid environment,
                and consist of alternating isocyano-terminated benzene monomers coordinated to gold
                atoms. We show that the chaining process is critically determined by the surface
                density of molecules. In particular, we demonstrate that by reducing the local
                supply of molecules within the junction, either by lowering the molecular
                concentration or by adding side groups, the oligomerization process can be
                suppressed. Our experimental results are supported by ab-initio simulations,
                confirming that the isocyano terminating groups display a high tendency to form
                molecular chains, as a result of their high affinity for gold. Our findings open the
                road for the controlled formation of one-dimensional, single coordination-polymer
                chains as promising model systems of organometallic frameworks. Highly-ordered systems combining metal and organic components have
                recently generated a considerable interest for applications in catalysis, storage
                and sensing applications. Two-dimensional metal-organic frameworks as electronic
                    systems [1] , [2] , [3] , [4] also raise increasing interest thanks to their
                appealing electric properties, such as high electron
                    mobilities [5] and very large volumetric and areal
                    capacitances [6] . Their one-dimensional counterparts may offer
                alternative routes for bottom-up nanoscale electronics [7] given the ability of the
                transition metal centers to change oxidation states and greatly enhance their
                ability to transport charge [8] . A distinct advantage of these hybrid
                organic–inorganic systems over all-organic polymers is that they typically do not
                require dopants to achieve charge transport. Such hybrid materials are typically
                prepared either by coordination chemistry or by solvo-thermal and hydro-thermal
                syntheses, providing only limited control over the dimension of the formed oligo-
                and/or polymers. Moreover, the large influence of the local environment on the chain
                conformations largely dominates the microscopic dynamics of the growth process,
                resulting in chain-to-chain variations of the length, tacticity and comononer
                incorporation. If such organometallic architectures are to play a role in nanoscale
                electronics, assembly at the single monomer level is crucial to achieve, as this
                will allow for an ultimate control over the chain composition and length. Step-by-step growth of polymers has been first monitored in a protein
                nanoreactor using spatially separated reactants [9] . Moreover, self-assembled
                monolayers have been used as a platform to create and control the formation of
                polymers by alternating precursor molecules [10] . More recently, controlled
                growth of a single polymer was achieved using magnetic
                    tweezers [11] . Supported by molecular dynamics, the growth
                dynamics, and in particular the incorporation of new monomers, was studied in
                detail, with polymer lengths up to several microns. Oligomerization has also been achieved in molecular devices by the
                incorporation of metal ions between receptor molecules connected to
                    metal [12] and graphene [13] electrodes or by means of click
                    chemistry [14] , [15] . However, in these cases the growth process was not monitored in real-time, and a
                stepwise addition of precursors was required. Moreover, the length of the chains was
                fixed in advance by the device geometry, and could therefore not be adjusted during
                the growth process. Finally, STM measurements on conjugated oligomers chains have been
                reported in which a chain is lifted up from the substrate using the STM
                    tip [16] , [17] , [18] , [19] . In these measurements however, the chains were already preformed on underlying gold
                the surface. The first signature of in situ dimerization in molecular junctions via
                covalent bonding was reported using the scanning tunneling microscope break-junction
                    technique [20] . However, no evidence for trimerization or
                higher-order oligomer formation has been reported. Here, we demonstrate the controlled formation, unit-by-unit, of single
                conductive coordination-oligomer chains, up to three units. Key to this achievement
                is the strong interaction of the isocyano groups with the gold electrodes which
                leads to a junction formation probability close to unity. This high affinity
                combined with the strongly dipolar nature of the isocyano anchor allow the molecules
                in a break junction system to form organometallic chains mediated by the
                incorporation of gold atoms. These atoms are provided by the electrodes, and do not
                require the stepwise addition of solutions or precursors. The chains are formed
                using mechanically controllable break junctions (MCBJ), and the chain formation is
                monitored in real-time by means of electrical characterization. Electrical characterization We perform electrical conductance measurements on the three
                  1,4-benzenediisocyanide derivatives displayed in Fig. 1a (abbreviated with: BdNC: 1,4-diisocyanobenzene; MBdNC:
                  1,4-diisocyano-2,5-dimethylbenzene; tBuBdNC: 1,4-diisocyano-2,5-di- tert -butylbenzene) using the MCBJ approach in liquid
                      environment [21] , of which a schematic layout is depicted in
                    Fig. 1b . In this technique, a
                  nanometer-sized gold wire is broken in the presence of the molecular solution. Upon breaking the gold wire forms atomically sharp electrodes, which the molecules
                  can bridge. After breaking of the gold-molecule junction, the gold contacts are
                  fused again and the process is repeated, allowing to address many different
                  junction configurations. Throughout the entire opening/closing cycle, the current
                  through the junction is monitored. The calibration of the distance is performed as
                  described previously [21] . The measurements are performed at room
                  temperature in 100 μM solution in a 1:4 (v/v) mixture of tetrahydrofuran (THF) and
                  mesitylene (Mes) as solvent. More details concerning the experiments are described
                  in the Methods section. Fig. 1 Double plateau formation in isocyano compounds. a Structural formula of measured compounds. b Schematics of MCBJ setup for liquid
                          measurements. c Overview of BdNC
                          measurements: 1445 opening conductance traces at 0.1 V bias voltage in
                          100 μM solution in THF:Mesitylene 1:4 (v/v). Central panel:
                          conductance-displacement histogram and two typical opening traces. The
                          histogram displays the counts per bin on a linear scale with 25 bins per
                          decade of conductance and a bin size of 0.15 Å for displacement. Sample
                          traces are shifted horizontally for clarity. Right panel: conductance
                          histogram with 25 bins per decade. Red dashed curves represent Gaussian
                          fit of the conductance peaks. d Overview
                          of closing traces analysis: 1445 traces at 0.1 V bias voltage in 100 μM
                          BdNC solution. Central panel: conductance-displacement histogram and two
                          typical closing traces. Right panel: conductance histogram with 25 bins
                          per decade; red curve: conductance histogram of opening traces shown in
                            ( c ) Full size image Measurements on BdNC The central panel of Fig. 1c displays two representative breaking traces recorded on the BdNC molecule,
                  alongside the corresponding conductance-displacement histogram, built from 1445
                  breaking traces recorded on 6 different samples at a bias voltage of 0.1 V and
                  without any data selection. All breaking traces are aligned in displacement at the
                  rupture point of the last gold–gold contact. As a prominent feature in the
                  conductance-displacement histogram we observe the formation of two plateau-shaped
                  regions of high counts, one at high conductance (plateau 1, abbreviated as P1) and
                  one at low conductance (plateau 2, abbreviated as P2). We also note that a
                  prominent peak is visible at 1 G 0 , and very few counts down
                  to the P1 plateau, indicative of atomically sharp electrodes. In between the two
                  plateaus, abrupt jumps in conductance are observed, as is apparent from the
                  individual breaking traces. After P2, no distinct region of high counts is present
                  down to the noise floor of our measurement setup, which is around
                    2 × 10 −6 G 0 . The most probable
                  conductance value of each plateau is obtained by fitting the two peaks in the
                  conductance histogram to Gaussian distributions, as illustrated in the right panel
                  of Fig. 1c . The fitted conductance values
                  are G P1 = 10 −2.1 G 0 = 8 × 10 −3 G 0 and
                    G P2 = 10 −3.7 G 0 = 2 × 10 −4 G 0 for the P1 and P2 plateau, respectively. Another
                  remarkable observation is that the yield of junction formation is more than 99%
                  (see Supplementary Note 1 for more
                  details). This value is high for molecular junctions, even for liquid
                      environments [22] . BdNC molecules were previously measured in self-assembled
                      monolayers [23] , in MCBJ setup at cryogenic temperatures in high
                      vacuum [24] and using the scanning tunneling microscopy
                  break junction (STM-BJ) approach in solution [25] , [26] , [27] . In none of those
                  measurements the formation of two conductance plateaus was reported. However, the
                  P2 plateau in our experiment appears at a conductance lower than the detection
                  limit ( G > 10 −4 G 0 ) of the latter study. More generally speaking, the
                  presence of multiple conductance plateaus or multiple conductance peaks has been
                  observed previously for other molecules and was attributed to multiple molecules
                  in parallel bridging the electrodes [28] , [29] , multiple binding configurations of a single
                      molecule [30] , [31] , [32] , [33] , switching between internal conductance
                      states [24] , [34] , π – π -stacking [35] or rectification [36] with a different conductance
                  for the forward and reverse current direction. One way to distinguish between these scenarios is by comparing the
                  length of the breaking traces to the length of the molecule. To extract this
                  plateau length from the opening traces, we developed a plateau detection scheme of
                  which more details can be found in Supplementary Note 2 . From this analysis, we obtain an average length for the first
                  and second plateau of 6.4 and 9.0 Å, respectively. Including the retraction of the
                  electrodes of about 5 Å [22] , this observation suggests a total electrode
                  separation of about 20 Å at the end of the plateau P2. BdNC has a computed length
                  of 7.8 Å; scenarios involving multiple molecules in series are therefore more
                  feasible than those with a single molecule possessing multiple degrees of freedom
                  binding to the two electrodes (different ground/excited states, different binding
                  geometries, rectification). Closing traces analysis In order to gain more insight in the nature of the P2 plateau, we
                  also investigated the junction behavior upon closing of the gap between the
                  electrodes. Closing conductance traces have not been widely studied since for most
                  molecules no clear conductance features are observed [37] , [38] , [39] . This is usually attributed
                  to the fact that molecules tend to lay flat on the electrode surface after the
                  breaking of the molecular junction. 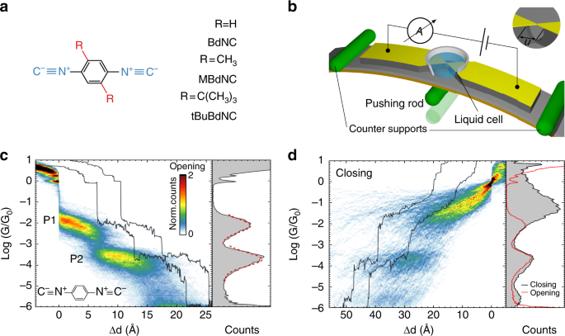Fig. 1 Double plateau formation in isocyano compounds.aStructural formula of measured compounds.bSchematics of MCBJ setup for liquid
                          measurements.cOverview of BdNC
                          measurements: 1445 opening conductance traces at 0.1 V bias voltage in
                          100 μM solution in THF:Mesitylene 1:4 (v/v). Central panel:
                          conductance-displacement histogram and two typical opening traces. The
                          histogram displays the counts per bin on a linear scale with 25 bins per
                          decade of conductance and a bin size of 0.15 Å for displacement. Sample
                          traces are shifted horizontally for clarity. Right panel: conductance
                          histogram with 25 bins per decade. Red dashed curves represent Gaussian
                          fit of the conductance peaks.dOverview
                          of closing traces analysis: 1445 traces at 0.1 V bias voltage in 100 μM
                          BdNC solution. Central panel: conductance-displacement histogram and two
                          typical closing traces. Right panel: conductance histogram with 25 bins
                          per decade; red curve: conductance histogram of opening traces shown in
                            (c) Figure 1d displays the
                  closing conductance traces acquired in the same experiment as Fig. 1c , presented in a similar fashion as the their
                  corresponding breaking traces, and aligned at 1 G 0 . Similar
                  to the breaking, two regions of high counts appear, with a large jump in
                  conductance in between them. Overall, two jumps in conductance are observed: the
                  first one is from the noise level of the setup to an intermediate state with a
                  conductance value close to G P2 . Here a plateau-like feature
                  is observed, followed by another jump in conductance to a second region of high
                  counts, ranging upwards from the P1 region of the breaking and slanted upwards. For comparison, the breaking histogram is plotted in red on top of the closing
                  histogram in the right panel of Fig. 1d . The P1 peak has a higher conductance and a larger width during the closing. This
                  effect is attributed to the evolution of the electrodes shape through an
                  opening/closing cycle; the electrodes are atomically sharp during opening and more
                  blunt during closing [37] . This is a result of the surface relaxation
                  after the breaking of the molecular junction, and least to more molecules bridging
                  the electrodes during closing. The P2 peak, on the other hand, has a similar
                  position, width, and height for both histograms, suggesting comparable junction
                  geometries are being probed. Moreover, upward jumps in conductance are visible,
                  both before and after the P2 plateau. This observation is remarkable, and uncommon for single molecule
                  measurements. The highly reproducible nature of the P2 plateau, combined with its
                  total length close to 20 Å suggests a strong type of interaction between the
                  molecules in series, while π – π -stacking is weak [35] , [40] . The binding energies for π – π -stacked molecule
                  are typically in the range of 10–100 meV, the same order of magnitude as k B T at room
                  temperature, making this type of interaction unlikely to yield such reproducible
                  conductance traces. In the following, based on theoretical calculations, we will
                  show that these distinct features, in fact, are indicative of the in situ
                  formation of molecular dimers. Theoretical calculations For further insights into the dynamics throughout the
                  opening/closing cycles, we have performed Density Functional Theory based
                  Molecular Dynamics (DFT-MD) simulations at room temperature of several molecular
                  junctions formed by BdNC molecules between gold electrodes using the codes
                      SIESTA [41] and GOLLUM [42] . For a detailed description
                  of these calculations, we refer to Supplementary Note 7 . In short, the electrodes are pulled apart in steps of 0.1 Å,
                  similar to the method reported previously [43] . The entire system is relaxed
                  by taking 200 DFT-MD steps of 1 fs each after each of those pulling steps. Each of
                  these DFT-MD steps is in turn accomplished as follows: the free energy of the
                  whole system at the desired temperature is calculated using DFT. The force felt by
                  each atom in the system is computed by direct differentiation of the above free
                  energy with respect to the atom displacements. Each atom is moved by solving
                  Newton’s classical equations of motion. The whole system is kept at the desired
                  target temperature using a Nose thermostat. Using this approach we have computed several opening and closing
                  traces of which snapshots are shown in Fig. 2a,
                    c , respectively. From these trajectories, two observations can be
                  made. First, we find that for electrode separations of up to 8 Å after the gold
                  neck is broken, a single molecule bridges the two electrodes, while for larger
                  separations the molecules tend to form a dimer chain. In fact, we find that BdNC
                  molecules have a strong tendency to polymerize in situ during the opening of the
                  junction. Moreover, the formation of these chains is always mediated by gold atoms
                  that are pulled out of the electrodes and are being inserted between the BdNC
                  monomers. In contrast, bare isocyano end-groups repel each other due to strong
                  Coulomb interaction of terminal carbon atoms of
                      isocyano-group [44] . Second, the BdNC molecules also tend to remain
                  perpendicular to the gold surface, rather than laying flat on the
                    electrodes. Fig. 2 Molecular dynamics simulation demonstrating chaining mechanism. a , c Snapshots of the molecular dynamics simulations for the opening and the
                          closing of the BdNC molecular junction, respectively, demonstrating the
                          chaining effect in presence of extra BdNC molecule. b , d Reconstructed
                          conductance traces along the corresponding DFT-MD trajectories. Numbered
                          points correspond to the snapshots in ( a , c ) Full size image To rationalize these observations, we performed additional
                  angle-dependent DFT-based total energy calculations (see Supplementary
                    Note 8 ). These calculations reveal the
                  highly directional nature of the isocyano–Au bond, that possesses a local energy
                  minimum for a contact angle of 90 degrees, in addition to the usual minimum at 0
                  degrees. We stress that the minimum at 90 degrees is absent for other molecules
                  like 1,4-benzenedithiol or 1,4-dicyanobenzene. This predisposition for large
                  contact angles results in a high packing density of the molecules on the electrode
                  surface with the molecules pointing with one side away from the electrodes. Combined with the very strong binding energy of the isocyano group to the gold,
                  this directionality allows us to rationalize the high yield of molecular junction
                  formation observed in the experimental data. Large binding energies are also known to promote the extraction of
                  gold atoms from the electrodes. Previous studies on electromechanical properties
                  of molecular junctions have shown that during the breaking of a molecular
                  junction, Au–Au bonds can be broken in the presence of a strong covalent bond
                  between the anchoring group (such as thiols) and gold
                      atoms [45] , leading to the pulling of atoms from the
                  electrodes. Another important aspect is that, due to Coulomb repulsion of terminal
                  C atoms, isocyano groups cannot bind directly to other isocyano groups. This
                  particularity therefore makes the formation of an organometallic chain the most
                  plausible scenario and is in line with gold-mediated isocyanide-based
                  organometallic compounds which have been observed in early crystallography
                      studies [46] , [47] and have more recently been synthesized and
                  studied in monolayers [48] . Based on the DFT-MD trajectories, we also computed the conductance
                  through the molecular junction as a function of electrode separation (for more
                  detailed information, see Supplementary Notes 9 and 10 ). The
                  resulting conductance traces are presented in Fig. 2b,
                    d for opening and closing of the electrodes, respectively. 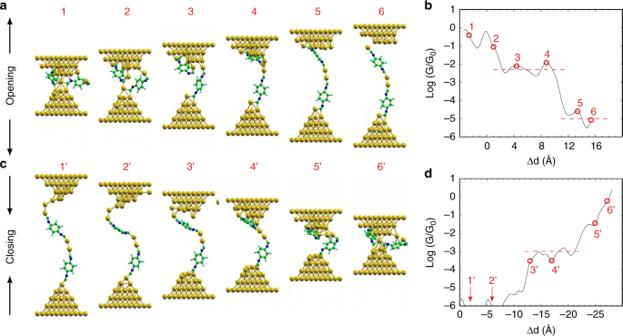Fig. 2 Molecular dynamics simulation demonstrating chaining mechanism.a,cSnapshots of the molecular dynamics simulations for the opening and the
                          closing of the BdNC molecular junction, respectively, demonstrating the
                          chaining effect in presence of extra BdNC molecule.b,dReconstructed
                          conductance traces along the corresponding DFT-MD trajectories. Numbered
                          points correspond to the snapshots in (a,c) For the
                  opening trace, shown in Fig. 2b , two
                  plateaus are visible. The first has a length of about 5 Å and a conductance of
                  about 5 × 10 −3 G 0 , while the
                  second one has a conductance of about 10 −5 G 0 . We note that the difference in conductance between
                  the two plateaus is more than two orders of magnitude. For the closing trace, we
                  find a 10 Å-long plateau with a conductance of about
                    10 −3 G 0 . We have performed 30 such opening traces (see Supplementary
                    Note 11 for more detail), 16 of which
                  ended in the successful formation of a molecular junction. This yield is lower
                  than in the experiments but one should keep in mind that the stretching speed of
                  the MD simulations is much quicker than the experimental one, and that no solvent
                  is present in the calculations, which may reduce the probability of the
                  oligomerization process to occur. Of these molecular junctions, 0 showed the
                  formation of a monomer, while in 5 a dimer was observed. Finally, one trace
                  yielded a monomer and a dimer in parallel, and we count this as a monomer because
                  the two compounds bridge the electrodes in parallel, bringing the total count of
                  monomer traces to 11. A conductance histogram is presented for both scenarios in
                    the Supporting Information . We find
                  that the histogram of the dimers agrees well with the experimental values of P1
                  and P2 of BdNC at high concentration. Moreover, the conductance histogram for the
                  simulated monomers resembles the experimental one for BdNC at low molecule
                  concentration. Altogether, the combined results of the DFT-MD simulations and NEGF
                  calculations are in line with experimental data, and point towards a chaining
                  model as most plausible explanation for the formation of the P2 plateau. Indeed,
                  the model provides a justification for the experimental traces being more than
                  twice as long as the length of the molecule by means of incorporating one or two
                  gold atoms during the formation of the organometallic dimer. Oligomerization Based on the high affinity of isocyanides to form organometallic
                  dimers, we expect the formation of oligomeres with a larger amount of repeating
                  units, such as trimers or tetramers to be plausible. In Fig. 1c , however, no signature for such events are
                  observed, and one may argue that this is either caused by their conductance being
                  below the noise floor of the setup, or their yield being too low to show up in the
                  conductance-displacement histogram. Based on the conductance of plateau P1 and P2,
                  and assuming an exponential dependence of the conductance on the amount of the
                  units, the conductance of the organometallic BdNC trimers is expected to be around G P 3 ≈ 10 −5.3 G 0 , and 10 −6.9 G 0 for tetramers. While the conductance of the tetramer
                  is outside our experimentally accessible conductance range, the one for the trimer
                  lays well within. To investigate this scenario and determine the cause for the
                  apparent lack of a third region of high counts, we developed a data filtering
                  scheme to identify plateaus in the conductance region where the trimers are
                  expected be present. For more information about this analysis scheme, we refer to
                  Supplementary Note 3 . By applying this
                  selection method on the data shown in Fig. 1 , 420 opening conductance traces (29%) were tested positively
                  for the presence of a third plateau. The conductance- and conductance-displacement
                  histograms of the corresponding traces are shown in Fig. 3a , together with a typical conductance trace. The
                  conductance-displacement histogram of selected traces exhibits three
                  plateau-shaped regions of high counts, arranged in a stair-like fashion, with
                  lengths of 6.4, 8.4 and 3.4 Å, respectively. The three areas of high counts yield
                  distinct peaks in the conductance histogram with conductance values, determined
                  from Gaussian fits, of
                    7 × 10 −2 G 0 ,
                    1.6 × 10 −4 G 0 and
                    5.0 × 10 −6 G 0 , respectively. The conductance decreases exponentially, with a decay constant of 1.56 decade per
                  unit. The remaining 1025 traces that were not selected (71%) are presented as an
                  inset in Fig. 3a . Here, in contrast, only
                  two plateaus are visible, with a clear drop in conductance after the breaking of
                  the second plateau. The ability of gold-capped BdNC molecules to form trimer
                  chains is confirmed by several MD-DFT simulations that we have carried out in
                  presence of simplified gold electrodes. Fig. 3 Observation of trimer formation. a Combined 2D–1D histogram and sample trace for 420 opening
                          conductance traces (29%) for 100 μM BdNC measurements exhibiting third
                          plateau formation. Red curves represent Gaussian fit of the conductance
                          histogram for the plateaus yielding conductance values of
                            7 × 10 −2 G 0 ,
                            1.6 · 10 −4 G 0 and
                            5.0 × 10 −6 G 0 for
                          plateaus P1, P2 and P3, respectively. 2D–1D histogram for remaining 1025
                          traces (71%) is shown on the inset. b Experimental and computed conductance decay versus number of BdNC units. Error bars correspond to the standard deviations of the conductance peaks
                          fit in ( a ). c The three junction geometries containing one gold atom as
                          interconnect that have been used to compute the transmission shown in
                            ( d ). 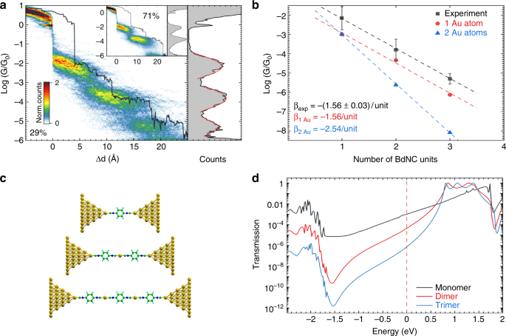Fig. 3 Observation of trimer formation.aCombined 2D–1D histogram and sample trace for 420 opening
                          conductance traces (29%) for 100 μM BdNC measurements exhibiting third
                          plateau formation. Red curves represent Gaussian fit of the conductance
                          histogram for the plateaus yielding conductance values of
                            7 × 10−2G0,
                            1.6 · 10−4G0and
                            5.0 × 10−6G0for
                          plateaus P1, P2 and P3, respectively. 2D–1D histogram for remaining 1025
                          traces (71%) is shown on the inset.bExperimental and computed conductance decay versus number of BdNC units.
                          Error bars correspond to the standard deviations of the conductance peaks
                          fit in (a).cThe three junction geometries containing one gold atom as
                          interconnect that have been used to compute the transmission shown in
                            (d).dCalculated transmission functions for the chains formed by 1–3 BdNC units
                          with one gold atom between units d Calculated transmission functions for the chains formed by 1–3 BdNC units
                          with one gold atom between units Full size image Figure 3b shows the
                  extracted conductance value as a function of the number of units present in the
                  chain, following an exponential decay of −1.56 decade per unit. To rationalize
                  this trend, we have computed the conductance of BdNC–Au oligomer chains with up to
                  three repeating units using SIESTA and GOLLUM, for the cases where one and two
                  gold atoms interconnect the BdNC units. Figure 3c presents the junction geometries for the monomer, dimer, and
                  trimer chains having one interconnected Au atom, and Fig. 3d displays the respective transmission curves. We
                  refer to the Supplementary Note 13 for
                  the figures corresponding to two inter-connecting gold atoms. The computed
                  transmissions decays are −1.56 and −2.54 for the two cases, respectively. This
                  observation suggests that the monomers may be interconnected by one gold atom, in
                  agreement with the geometry of previously observed
                      complexes [44] . Surface coverage study With the formation of the second and third plateau understood in
                  terms of a chaining effect, the next step is to understand and control the
                  formation of these chains. For chains to form in a repeatable manner, a supply of
                  molecules is required. The dynamics of the chaining process is therefore expected
                  to be determined by the proximity of other molecules, i.e., it should depend on
                  the surface coverage of the electrodes. To investigate the role of the molecular
                  coverage, we employed two approaches. In the first approach, the coverage is
                  influenced by varying the concentration of the molecular solution in which the
                  measurements are performed. In the second one, side groups promoting steric
                  hindrance are added to the molecule. To investigate the influence of the concentration, we studied the
                  molecular junction formation in solutions with 10 nM and 1 μM concentrations. The
                  first observation is that the signature of the molecular junction formation is
                  distinctively different for each concentration regime, as can be seen in the
                  conductance and conductance-displacement histograms of the corresponding figures
                  (see Fig. 4a, b, d ). For a 10 nM
                  concentration, only one slanted conductance plateau is observed, resulting in a
                  peak at G ≈ 10 − 3.1 G 0 = 8 × 10 −4 G 0 , with a ≈93% junction formation probability. This
                  conductance value is close to the one reported for BdNC molecules in STM-BJ
                      measurements [26] , [27] . We therefore attribute this plateau to a
                  single- or few-molecule configuration. For the 1 μM solution, the plateau is less
                  slanted and appears at a conductance value of 10 −2.3 G 0 = 5 × 10 − 3 G 0 with a higher yield of
                  99%. For a 100 μM solution, Fig. 4a shows
                  the two previously observed plateaus. Finally, to highlight the role of the
                  molecule supply, we also performed measurements in dry conditions (see
                  Supplementary Note 6 ), in which case
                  very few molecules are expected to be available for the oligomerization process. This rationale is indeed confirmed by the reported measurement which do not show
                  the formation of a dimer but rather a single conductance peak. Fig. 4 Concentration and steric hindrance effect on the chain
                          formation. Combined 2D–1D histograms for ( a ) 100 μM BdNC solution measurement (1445 traces), lower
                          concentration measurements: b 1 μM BdNC
                          solution (350 traces), d 10 nM BdNC
                          solution (200 traces), and measurements for BdNC derivatives with side
                          groups: c 100 μM MBdNC (374 traces) and
                            ( e ) 100 μM tBuBdNC solution (565
                          traces). Typical opening conductance trace is shown for every
                          measurement Full size image The second method to tune the coverage is via steric hindrance. This is achieved by the addition of side groups, and for this purpose, we studied
                  two 2,5-disubstituted derivatives of BdNC: 2,5-dimethyl-1,4-benzenediisocyanide
                  (MBdNC, R=CH 3 ) and 2,5-di- tert -butyl-1,4-benzenediisocyanide (tBuBdNC,
                    R=C(CH 3 ) 3 ), with tBuBdNC being the
                  most bulky of the two. The bulky side groups of these molecules reduce the
                  proximity of neighboring molecules at the electrode surface and therefore the
                  availability of an additional molecule for chaining. All measurements were
                  performed in 100 μM solutions of THF:Mes mixture as before. In the case of MBdNC, we observe one plateau with a conductance
                  value, a peak shape and a plateau length very close to the P1 plateau of the BdNC
                  molecule (Fig. 4c ). The yield of junction
                  formation is almost 100%. For the tBuBdNC molecule, only one short and slanted
                  conductance plateau ( G ≈ 5 × 10 −4 G 0 )
                  is observed with a lower yield of 91.3% (Fig. 4e ). Qualitatively, the signatures of the molecular junction
                  formation for MBdNC and tBuBdNC resemble the ones obtained for the 1 μM and 10 nM
                  solutions of BdNC, respectively. Overall, both the concentration and the side group study
                  demonstrate that the molecular coverage of the electrode surface is of paramount
                  importance for the formation of the P2 and P3 plateau, i.e., chaining is only
                  possible when additional molecules are sufficiently closeby at the moment the
                  molecular bridge breaks. Plateau analysis Another interesting observation from Fig. 4 is that the molecular supply not only affects the
                  polymerization process, but also the shape of the P1 conductance plateau. The
                  influence of the coverage on the plateau shape may shed some light on the
                  dynamics, and for this purpose we performed an additional shape analysis of
                  plateau P1 for the various molecules and concentrations in order to quantify the
                  plateau width, slope, and center (see Supplementary Note 4 for more details). Determining the plateau
                  properties was done by fitting the areas of high counts in the
                  conductance-displacement histograms with two-dimensional Gaussians, as illustrated
                  in Fig. 5a . The extracted values are shown
                  in Fig. 5b . The plot shows that both the
                  plateau width and slope monotonously decrease with increasing concentration and
                  decreasing side group size, while the center, on the other hand, moves towards
                  higher conductance values. Fig. 5 Analysis of conductance plateaus. a Schematics of plateau shape analysis for 100 μM BdNC
                          measurements. b Plateau width, center and
                          slope deduced from the shape analysis (see Supplementary Note 4 for more details). c Schematic sketch of the possible scenario’s for different
                          surface coverages. Molecules connected to both electrodes are depicted in
                          red, while the others are colored gray Full size image The apparent similarity of the plateaus is confirmed by a
                  calculated correlation of the plateau properties for the two different approaches
                  for tuning the surface coverage (0.997, 0.964, and 0.9997 for the width, slope,
                  center, respectively). This correlation motivates us to search for a single
                  mechanism to explain the data from both approaches. The observed changes in
                  junction formation with surface coverage shown in Fig. 5b can be rationalized by considering the role of inter-molecular
                  interactions. Let us first focus on the plateau width. The reduction in plateau
                  width is a result of a decrease in conductance fluctuations within each
                  conductance trace (see Supplementary Note 5 ), and is indicative for the formation of more stable molecular
                  junction. This most likely results from a reduction of mechanical degrees of
                  freedom due to the formation of molecular stacks composed of a few molecules
                  bridging the electrodes in parallel. One can argue along similar lines when
                  considering the downward orientation of the plateaus. The pronounced slope may be
                  due to sliding of a single molecule on the electrodes during opening of the
                  junction, the probability of which is being reduced when decreasing the number of
                  mechanical degrees of freedom when forming molecular stacks. This hypothesis
                  concerning the formation of stacks is corroborated by the upwards shift in the
                  center of the plateaus with increasing coverage, a signature of parallel
                  conduction though an increased number of molecules. These scenarios are
                  schematically depicted in Fig. 5c . For low
                  and medium coverage, only single, or few molecules bridge the gap, while for high
                  densities molecular stacks are formed for small electrode separations, followed by
                  dimers and trimers upon increase of the electrode spacing. It is important to keep in mind that the high molecular coverage is a
                result of the directionality of the isocyano–Au bond, as it allows for densely
                packed arrays of molecules. This density is determined by the concentration of
                molecules in solution. For high coverages, this results in the formation of dimers
                and trimers, suggesting the experimental conditions play a crucial role in the
                polymerization process. This strict criterium may explain why previous studies have
                not observed this chaining phenomenon, as measurements were either performed in dry
                conditions, or at lower concentrations. Another point which should be noted is that the formation probability
                of trimers of 29% may be increased by performing the measurements in a molecular
                solution of higher concentration. However, this approach has as drawback that for
                high surface coverages, the junction tends to have difficulties closing to full
                contact, thereby severely limiting the number of opening traces which can be
                acquired on a junction. In the present study, the metallic atoms to form the
                coordination-oligomer chains were provided by the electrodes by means of extraction
                during the opening of the junction. This conclusion is supported by the lack of the
                P2 plateau at low concentrations, which would be present in case the in-solution
                formation of Au-mediated dimers would play a role. Alternatively, one could also
                engineer the junctions such that the metallic atoms are supplied by ions present in
                solution. This approach would allow for more flexibility in terms of available metal
                centers, and for instance allow to incorporate magnetic atoms for spintronics
                studies in metalorganic spin-chains, while keeping the convenience of gold
                electrodes for contacting the chains. Finally, our approach for high surface
                coverage may be more widely exploited for the realization of mechanically
                stabilizing molecular junctions, both with the prospect of reducing electronic
                variability, as well as increasing the robustness in terms of electrode
                separation. In summary, we demonstrate the controlled formation of organometallic
                oligomer chains in solution up to three repeating units. This is achieved by
                utilizing isocyano anchoring groups, which combine a highly directional binding with
                a strong binding energy. The anisotropic binding allows for high surface coverages
                and yield of junction formation, while the strong binding leads to the extraction of
                gold atoms from the electrodes, thereby acting as supply of metal ions. We show that
                the formation of such coordination-oligomer chains can be affected by varying the
                molecular supply, either by reducing the concentration of molecules, or by the
                addition of steric side-groups. The influence on the molecular supply provides
                insights in the formation process of the molecular junctions and points towards the
                formation of molecular stacks of several molecules in parallel. 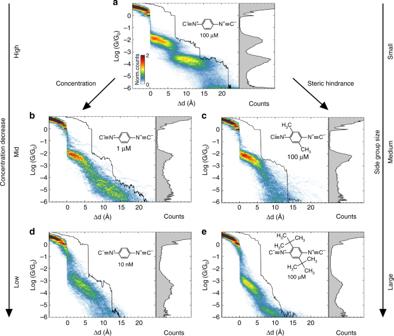Fig. 4 Concentration and steric hindrance effect on the chain
                          formation. Combined 2D–1D histograms for (a) 100 μM BdNC solution measurement (1445 traces), lower
                          concentration measurements:b1 μM BdNC
                          solution (350 traces),d10 nM BdNC
                          solution (200 traces), and measurements for BdNC derivatives with side
                          groups:c100 μM MBdNC (374 traces) and
                            (e) 100 μM tBuBdNC solution (565
                          traces). Typical opening conductance trace is shown for every
                          measurement 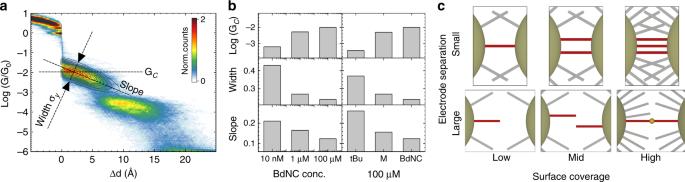Fig. 5 Analysis of conductance plateaus.aSchematics of plateau shape analysis for 100 μM BdNC
                          measurements.bPlateau width, center and
                          slope deduced from the shape analysis (see Supplementary Note4for more details).cSchematic sketch of the possible scenario’s for different
                          surface coverages. Molecules connected to both electrodes are depicted in
                          red, while the others are colored gray Our findings are
                supported by DFT + NEGF calculations, demonstrating both the crucial role of the
                anisotropic binding, as well as the importance of the metal ions in the chain. An
                interesting side-effect of the high packing density is the reduction of fluctuations
                in junction conductivity Conductance histograms The experiments are performed using the mechanically-controllable
                  break-junction (MCBJ) approach in solution at room temperature. The MCBJ samples
                  were fabricated as described previously [35] . In short, a suspended gold bridge of about
                  500 to 700 nm was fabricated with a 60 nm wide constriction in the center, for a
                  film thickness of 60 nm. To reduce parasitic currents in liquid, an additional
                  layer of 3 μm thickness of photodefinable polyimide was deposited to cover the
                  electrodes, while keeping the gold bridge itself exposed. All molecular solutions
                  were freshly prepared for each measurement using the mixture of THF and Mes (ratio
                  1:4 v/v) as a solvent. For each sample, the gold bridge was initially broken in
                  pure solvent and 50 opening-closing cycles were recorded. After that, the liquid
                  cell was filled with the target molecular solution. For every cycle, the junction
                  was opened until the conductance of 10 −6 G 0 (noise level of the setup) was reached, followed by a
                  subsequent closing of the gold contact (~10 G 0 ). The speed
                  of the pushing rod was set to 31.2 μm/s. The measurements were performed with a
                  sampling rate of 500 Hz and a bias voltage of 0.1 V. The obtained opening and
                  closing traces were analyzed without any data selection. Opening traces were aligned at the breaking of the last atomic gold
                  contact. Conductance histogram and conductance-displacement histogram were build
                  by bining the opening traces both in distance and in conductance on log scale,
                  using 67 bins per nanometer and 25 bins per decade of conductance. The number of
                  counts then was normalized by the number of traces and sizes of the bins. Due to
                  discreteness of the analogue to digital converter and log-conversion, a few
                  artifacts (spikes in conductance histogram and stripes in conductance-displacement
                  histogram) occur for the conductances below 10 −5.5 G 0 . The closing conductance traces are treated as
                  reversed opening traces and analyzed in the same way. To build
                  conductance-displacement histogram for the closing traces, the traces were aligned
                  at the point with the conductance of G 0 .